Dynamic competition between spin-density wave order and superconductivity in underdoped Ba1−xKxFe2As2 An intriguing aspect of unconventional superconductivity is that it always appears in the vicinity of other competing phases, whose suppression brings the full emergence of superconductivity. In the iron pnictides, these competing phases are marked by a tetragonal-to-orthorhombic structural transition and a collinear spin-density wave (SDW) transition. There has been macroscopic evidence for competition between these phases and superconductivity as the magnitude of both the orthorhombicity and magnetic moment are suppressed in the superconducting state. Here, using angle-resolved photoemission spectroscopy on detwinned underdoped Ba 1− x K x Fe 2 As 2 , we observe a coexistence of both the SDW gap and superconducting gap in the same electronic structure. Furthermore, our data reveal that following the onset of superconductivity, the SDW gap decreases in magnitude and shifts in a direction consistent with a reduction of the orbital anisotropy. This observation provides direct spectroscopic evidence for the dynamic competition between superconductivity and both SDW and electronic nematic orders in these materials. To understand the phenomenon of high-temperature superconductivity (HTSC), it is important to understand the competing states of the superconducting phase. In both families of HTSC materials, the competing states consist of various symmetry-breaking phases, which interact with superconductivity (SC) in intricate ways. In the cuprates, one of the biggest puzzles is the nature of the pseudogap (PG) phase, which envelops a large portion of the superconducting dome in the phase diagram. Recently, a large amount of experimental evidence suggests a competition between the PG and SC [1] , [2] , [3] , [4] . However, the controversial nature of the PG phase itself complicates a direct study of this competition. Conversely, in the iron pnictides, the competing phases are well characterized: a collinear spin-density wave (SDW) order has been well established as the main competing phase in the underdoped (UD) region of iron pnictides [5] , [6] , while a nematic phase associated with the structure transition ( T S ) has been suggested as another competing phase [7] , [8] , [9] , [10] , [11] . The two transitions associated with these competing orders track each other closely, occurring either simultaneously or with T S preceding T SDW . SC emerges as these phases are suppressed with carrier doping, isovalent substitution, or pressure [12] , [13] . The way in which these two orders interact with SC varies among the pnictide families: while SC and SDW exhibit mutual exclusion in the Ln FeAsO families [14] , there is a large region of coexistence in both the NaFeAs [15] and the BaFe 2 As 2 families [16] , [17] , [18] . In addition, transport and neutron scattering experiments have shown that the orthorhombicity and magnetic moment, which are the macroscopic order parameters for the structural and SDW orders, are suppressed with the onset of SC [19] , [20] , [21] , signalling macroscopic competition between these orders and SC. In this paper, we focus on the phase competition between these orders and SC, which makes UD Ba 1− x K x Fe 2 As 2 in the coexistence region an ideal candidate as T S / T SDW and T C are well separated; yet, T C is sufficiently high to be experimentally accessible [18] . In particular, we study the electronic structure of a UD compound ( x =0.15), where T S = T SDW =110 K and T C =14.5 K, and the non-superconducting undoped BaFe 2 As 2 compound ( x =0) with T S = T SDW =138 K for comparison. Using high-resolution angle-resolved photoemission spectroscopy (ARPES), we directly observe the electronic response of each order in this compound. Distinct spectral signatures of the three orders are observed to coexist on the same electronic structure below T C , signalling the microscopic coexistence of the three orders. More importantly, we observe the spectral gap associated with the SDW order to be suppressed with the onset of SC. Furthermore, using a tight-binding model, we show that a reduction in the nematic order parameter is also needed to fully account for the observed shift of the SDW gap below T C . These observations show a direct electronic competition between the SDW and nematic orders with SC in Ba 1− x K x Fe 2 As 2 . Spectral evolution across phase transitions The momentum-resolved electronic structure, which can be directly imaged by ARPES, is expected to undergo distinct changes at each of the transitions in the system. As illustrated in the generic schematic in Fig. 1b , starting in the normal state ( T > T S , T SDW ), the typical electronic structure of iron pnictides consists of hole bands at the Brillouin zone (BZ) centre, Γ point, and electron bands at the BZ corner, X point. Lowering the temperature approaching T S , orbital-dependent band shifts onset, as has been observed in Co-doped BaFe 2 As 2 (ref. 9 ) and NaFeAs [22] , where bands dominated by the d xz (d yz ) orbital character shift down (up) in a k -dependent fashion (minimal at Γ and maximal at X , see Supplementary Fig. 1 ; Supplementary Note 1 ), breaking C 4 rotational symmetry. Across T SDW , translational symmetry is broken and bands fold along Q SDW =(π,π), opening SDW gaps such that the Fermi surface reconstructs, leaving portions ungapped. Finally, as the system is cooled below T C , particle-hole symmetric superconducting gaps open on bands that cross the Fermi level, E F . Hence, there are distinct spectroscopic signatures associated with the three order parameters in this system. 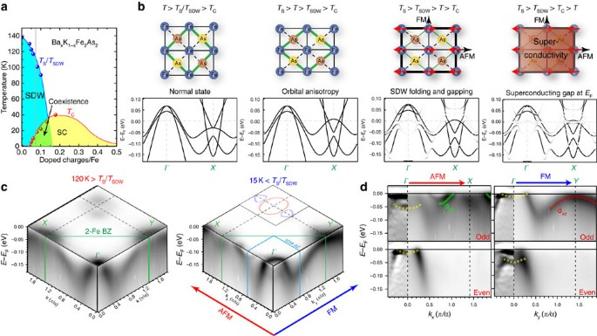Figure 1: Schematic and spectral evolution across phase transitions. (a) Phase diagram of Ba1−xKxFe2As2adapted from ref.18, where the grey vertical line indicates the doping of the UD compound studied. (b) Schematic of the expected evolution of the band structure acrossTS,TSDWandTC. From left to right, the four panels exhibit the band structure along the high-symmetry directionΓ–Xin the 2-Fe BZ, starting with the normal state (T>TS,TSDW), with the incremental addition of orbital anisotropy (TS>T>TSDW), SDW folding and gapping (TS/TSDW>T>TC) and finally SC (T<TC). (c) Measured electronic structure (Fermi surface and band dispersions) in the normal state and SDW state (belowTS/TSDWbut aboveTC) of the UD compound, with mixed even and odd light polarization. The reconstructed Fermi surface in the SDW state is outlined. (d) Band dispersions measured with purely even or odd polarization along the AFM and FM directions in the SDW state at 15 K. Thek<0 portions are second energy derivatives of the raw spectra. The hole-like band identified as dyzalong AFM and dxzalong FM are labelled, signalling the electronic nematicity. The electron bands folded from theXpoint to theΓpoint are marked with yellow dotted curves. All measurements were taken with 47.5 eV photons. Figure 1: Schematic and spectral evolution across phase transitions. ( a ) Phase diagram of Ba 1− x K x Fe 2 As 2 adapted from ref. 18 , where the grey vertical line indicates the doping of the UD compound studied. ( b ) Schematic of the expected evolution of the band structure across T S , T SDW and T C . From left to right, the four panels exhibit the band structure along the high-symmetry direction Γ – X in the 2-Fe BZ, starting with the normal state ( T > T S , T SDW ), with the incremental addition of orbital anisotropy ( T S > T > T SDW ), SDW folding and gapping ( T S / T SDW > T > T C ) and finally SC ( T < T C ). ( c ) Measured electronic structure (Fermi surface and band dispersions) in the normal state and SDW state (below T S / T SDW but above T C ) of the UD compound, with mixed even and odd light polarization. The reconstructed Fermi surface in the SDW state is outlined. ( d ) Band dispersions measured with purely even or odd polarization along the AFM and FM directions in the SDW state at 15 K. The k <0 portions are second energy derivatives of the raw spectra. The hole-like band identified as d yz along AFM and d xz along FM are labelled, signalling the electronic nematicity. The electron bands folded from the X point to the Γ point are marked with yellow dotted curves. All measurements were taken with 47.5 eV photons. Full size image To avoid twinning effects in the orthorhombic state, all measurements were performed on mechanically detwinned samples held under uniaxial stress. Although the effect of the detwinning stress on the transition temperatures has not been systematically studied in the Ba 1− x K x Fe 2 As 2 system, such a study in the Ba(Fe 1− x Co x ) 2 As 2 system shows that the stress naturally broadens T S to higher temperature [7] , but does not affect the full magnitude of the orbital anisotropy at the lowest temperature [9] ; ( Supplementary Note 1 ). Furthermore, in a systematic study in the BaFe 2 (As 1− x P x ) 2 system, it is shown that the mechanical detwinning stress increases T SDW and decreases T C (ref. 23 ). In the current study, we do not observe any significant modification of T SDW and T C within experimental uncertainties inferred from the temperatures at which spectral features associated with these orders onset compared with those measured on unstressed crystals. Figure 1c shows the changes observed across T S / T SDW for the UD sample. In the normal state, the Γ − X and Γ − Y directions are degenerate, respecting C 4 symmetry. Lowering temperature below T S / T SDW lifts this degeneracy, leading to the observed C 4 symmetry breaking. More specifically, measuring band dispersion with light polarized perpendicular to the cut direction ( Fig. 1d upper panels) reveals that the hole-like band with predominantly d yz character along the antiferromagnetic (AFM) direction near X moves to higher energy than the corresponding d xz band along the ferromagnetic (FM) direction near Y , a signature of the orbital anisotropy seen in the nematic phase of Co-doped BaFe 2 As 2 (ref. 9 ). In fact, the magnitudes of the orbital energy splitting in the K-doped samples are comparable to those in Co-doped samples, and roughly scale with T S independent of the type of doping ( Supplementary Fig. 2 ). Furthermore, electron bands folded from the BZ corner can be observed at the Γ point, indicative of long-range SDW order. These signatures of the nematic and SDW orders in the UD case are very similar to those observed in BaFe 2 As 2 , as a chemical potential shift of ~50 meV roughly mimics the doping effect between BaFe 2 As 2 and the UD sample ( Supplementary Note 1 ). SDW gaps open where the folded electron bands cross the hole bands near Γ ( Fig. 2 ). In BaFe 2 As 2 , the SDW gaps can be seen around −60 meV and −15 meV along those cuts ( Fig. 2a ). Focusing on the deeper SDW gap, the gap opens at T SDW and monotonically increases with lowering temperature as no other transitions exist below T SDW , similarly to the behaviour of the magnetic moment [20] , [21] . The more interesting case occurs in the UD compound, in which an SDW gap around −15 meV corresponds to the one discussed in BaFe 2 As 2 . 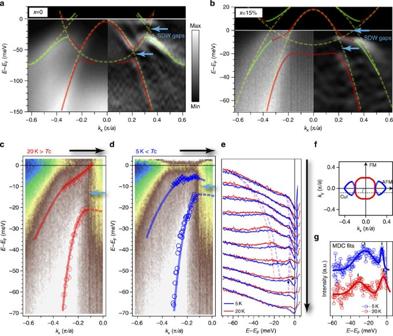Figure 2: Suppression of SDW gap belowTC. (a) Band dispersions of BaFe2As2measured in the SDW state (10 K) nearΓas labelled in (f). The left-hand side is the raw image, the right-hand side the second energy derivative. Guides to the eye for the dispersions are marked in colour, highlighting the dominant orbital character (red for dxz; green for dyz). As the dispersions are the result of SDW folding and gapping, the inferred bands before SDW gapping are marked by yellow dashed lines. (b) Same asabut for the UD (x=0.15) sample, measured in the SDW state aboveTCat 20 K. (c) The band dispersions frombnear the SDW gap taken aboveTC, divided by the Fermi-Dirac function convolved with a Gaussian representing instrument resolution. Open symbols are fitted peak positions of the energy distribution curves (EDCs) indicating the band dispersions. Blue arrow points to the SDW gap in discussion. (d) Same measurement but taken belowTC, at 5 K. (e) Comparison of EDCs taken aboveTC(red, 20 K) and belowTC(blue, 5 K) across the SDW gap in the momentum range marked by the black arrows in (c,d). Dashed lines trace out the band dispersions. Black circles highlight opening of the SC gap atkF. (f) Schematic of the reconstructed FS in the SDW state. (g) The momentum distribution curves of (c,d) are fitted with two Lorentzians and a linear background. The intensity of the inner hole band is plotted above (red) and below (blue)TC, where the separation of the two prominent peaks (black marks), measuring the effective SDW gap, shrinks belowTC. Measurements were taken with 25 eV photons. Figure 2c,d compare the evolution of this SDW gap above (20 K) and below (5 K) T C , where the bands forming the gap are marked. Cooling the sample below T C , the SDW gap magnitude abruptly decreases, which can be better visualized in two ways. First, comparing the energy distribution curves (EDC) above and below T C ( Fig. 2e ), we see two changes: (i) at k F where the upper band crosses E F , a SC gap opens (circles); (ii) the lower band shifts up in energy (dashed curves), reducing the effective SDW gap size. Secondly, we can examine the momentum distribution curves, which are horizontal line cuts through the spectra images in Fig. 2c,d . We fit these momentum distribution curves with Lorentzians for the two hole bands ( Supplementary Note 2 ). As the bands are relatively steep, the fitted positions would trace out the underlying ungapped band dispersion, while the fitted intensity of the inner hole band would show a suppression within the energy range in which the SDW gap develops. The fitted intensity for the inner hole band is plotted in Fig. 2g for the two temperatures, where the separation between the two peaks is another measurement of the SDW gap, which clearly decreases below T C . Figure 2: Suppression of SDW gap below T C . ( a ) Band dispersions of BaFe 2 As 2 measured in the SDW state (10 K) near Γ as labelled in (f). The left-hand side is the raw image, the right-hand side the second energy derivative. Guides to the eye for the dispersions are marked in colour, highlighting the dominant orbital character (red for d xz ; green for d yz ). As the dispersions are the result of SDW folding and gapping, the inferred bands before SDW gapping are marked by yellow dashed lines. ( b ) Same as a but for the UD ( x =0.15) sample, measured in the SDW state above T C at 20 K. ( c ) The band dispersions from b near the SDW gap taken above T C , divided by the Fermi-Dirac function convolved with a Gaussian representing instrument resolution. Open symbols are fitted peak positions of the energy distribution curves (EDCs) indicating the band dispersions. Blue arrow points to the SDW gap in discussion. ( d ) Same measurement but taken below T C , at 5 K. ( e ) Comparison of EDCs taken above T C (red, 20 K) and below T C (blue, 5 K) across the SDW gap in the momentum range marked by the black arrows in ( c , d ). Dashed lines trace out the band dispersions. Black circles highlight opening of the SC gap at k F . ( f ) Schematic of the reconstructed FS in the SDW state. ( g ) The momentum distribution curves of ( c , d ) are fitted with two Lorentzians and a linear background. The intensity of the inner hole band is plotted above (red) and below (blue) T C , where the separation of the two prominent peaks (black marks), measuring the effective SDW gap, shrinks below T C . Measurements were taken with 25 eV photons. Full size image Model simulation To better understand this decrease in the SDW gap below T C , we have simulated the spectroscopic effects of three order parameters (Δ S , Δ SDW , Δ SC ) associated with the three transitions ( T S , T SDW , T C ) based on a five-orbital tight-binding model of BaFe 2 As 2 from density-functional theory (DFT) band structure [24] , which is shifted by 0.15 eV and renormalized by a factor of 3 to match the observed band structure for the UD compound. The order parameters are incorporated phenomenologically, with Δ S introduced as an orbital-dependent on-site energy shift between d xz /d yz that is momentum dependent (zero at Γ and maximal at X / Y ); Δ SDW as an interaction term in the orbital basis; and Δ SC as a particle-hole symmetric isotropic gap at E F . We examine the calculated band dispersions near Γ along the same cut as the data in Fig. 2c . 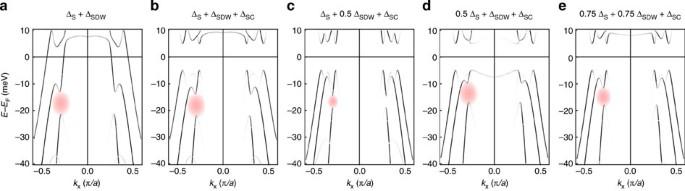Figure 3: Model simulation for the three order parameters. A tight-binding fit of BaFe2As2to DFT band structure is used, with a shift of 0.15 eV of the chemical potential and a renormalization factor of 3 to match the measured dispersion of the UD compound. The three order parameters are introduced phenomenologically to understand the effect on spectroscopy: (ΔS, ΔSDW, ΔSC, associated withTS,TSDW,TC). Calculations for the same cut as that inFig. 2are plotted here, with the SDW gap highlighted in pink. (a) Bands with only finite ΔSand ΔSDW, mimicking the situation in the orthorhombic SDW state aboveTC. (b) Simple addition of finite ΔSCwith no change in ΔSand ΔSDW, opening a SC gap atEF. The SDW gap is not much affected. (c) With addition of finite ΔSCand a reduced ΔSDW, the SDW gap size is reduced, but the centre does not shift. (d) With the addition of finite ΔSCand reduced ΔS, the effective SDW gap size is not much affected, but the gap centre shifts up. (e) When ΔSand ΔSDWare both moderately reduced, the effective SDW gap is both reduced in size and shifted up in energy, best matching the experimental observations. Figure 3a displays the situation deep in the orthorhombic SDW state but still above T C , with finite values for Δ S and Δ SDW . Here, we highlight in pink the SDW gap formed between the inner hole band and the folded electron band similar to the one observed experimentally in Fig. 2c . In the simplest scenario with no competition and SC added directly ( Fig. 3b ), only bands near E F are affected by the opening of a SC gap, with little effect on the observed SDW gap. In particular, the lower branch does not shift up, contrary to experimental observation. To account for the observed reduction in the SDW gap below T C , Δ SDW needs to be reduced before adding Δ SC ( Fig. 3c ). However, the centre of the gap does not shift noticeably relative to that above T C , whereas in the data, an overall shift towards E F is also observed in addition to the reduced gap size. To reproduce this shift, an additional reduction in Δ S is required ( Fig. 3d ). The best match to the experimental data is obtained by introducing a moderate reduction in both Δ SDW and Δ S ( Fig. 3e ). In reality, these two order parameters are intimately connected, as one enhances the other [25] , [26] , [27] . It is intrinsically difficult to separate these two effects, but the exercise displayed in Fig. 3 demonstrates the qualitative effects on the electronic structure of reducing each order parameter, and gives an intuitive understanding of the combined suppression of both orders below T C . Here, we note that the observed SDW gap shrinks in magnitude, as seen in the shift of the EDC peaks marking the boundary of the gap. This is the behaviour expected of the spectral evolution of a generic order parameter in competition. We note that our theoretical model here is based on an itinerant origin of the magnetism, while the general nature of magnetism in iron pnictides has not been fully settled, with proposals for coexistence of both itinerant and local magnetism [28] . In this regard, our observation of the reduction of the SDW gap itself shows a general competition of SC and SDW independent of the nature of the magnetism, as the gap size reflects the order parameter. The modelling presented here serves to demonstrate the effects of the competition on the electronic spectra. Figure 3: Model simulation for the three order parameters. A tight-binding fit of BaFe 2 As 2 to DFT band structure is used, with a shift of 0.15 eV of the chemical potential and a renormalization factor of 3 to match the measured dispersion of the UD compound. The three order parameters are introduced phenomenologically to understand the effect on spectroscopy: (Δ S , Δ SDW , Δ SC , associated with T S , T SDW , T C ). Calculations for the same cut as that in Fig. 2 are plotted here, with the SDW gap highlighted in pink. ( a ) Bands with only finite Δ S and Δ SDW , mimicking the situation in the orthorhombic SDW state above T C . ( b ) Simple addition of finite Δ SC with no change in Δ S and Δ SDW , opening a SC gap at E F . The SDW gap is not much affected. ( c ) With addition of finite Δ SC and a reduced Δ SDW , the SDW gap size is reduced, but the centre does not shift. ( d ) With the addition of finite Δ SC and reduced Δ S , the effective SDW gap size is not much affected, but the gap centre shifts up. ( e ) When Δ S and Δ SDW are both moderately reduced, the effective SDW gap is both reduced in size and shifted up in energy, best matching the experimental observations. Full size image Detailed temperature dependence Finally, we can trace the temperature-dependent evolution of this SDW gap by tracking the EDCs across the SDW gap ( Fig. 4a ), where the separation between the two peaks at each temperature represents the effective SDW gap magnitude. The SDW gap forms below T SDW , but instead of monotonically increasing with decreasing temperature as in BaFe 2 As 2 , it dips at the onset of SC ( Fig. 4c ). This behaviour is reminiscent of that of the orthorhombicity and magnetic moment observed in UD compounds [20] , [21] . To complete this comparison, we also plot the temperature dependence of the SC gap on the same inner hole band, which onsets at T C ( Fig. 4b,c ). Here, we note that the observed reduction in the SDW gap (~30%) seems much larger than that in the moment (~4%) for this doping [20] , [21] . The reason is that this observed decrease in the gap is actually a combined result of three effects: (i) opening of the SC gap pushing down the upper branch; (ii) reduction of Δ SDW ; and (iii) reduction of Δ S , which occur constructively at this particular momentum to magnify the effect. Depending on the precise interplay of these three ingredients, the overall effect at other momenta could be smaller, but the observed reduction in SDW gap is not limited to this momentum ( Supplementary Note 3 ). To further confirm such behaviour, we have performed mean-field calculations using tight-binding fits to the DFT-derived bands, including an ad-hoc isotropic SC order parameter and self-consistently determined orbital-dependent SDW. The results show that the introduction of SC indeed suppresses the SDW gaps, as naively expected from the usual interplay between SC and magnetism, where SC gaps quasiparticles around the Fermi surface, leaving much less spectral weight to simultaneously form the SDW order. The temperature dependence of the Δ SDW follows a trend similar to that shown in Fig. 4c ; ( Supplementary Note 4 ). 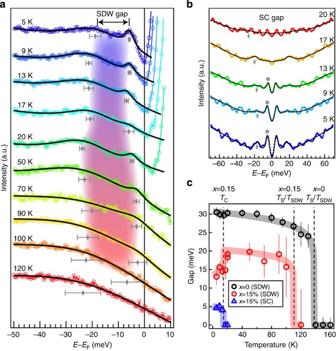Figure 4: Temperature dependence of the SDW and SC gaps. (a) EDCs divided by Fermi–Dirac function convolved with a Gaussian representing instrumental resolution taken across the SDW gap (integrated EDCs within a Δkx=0.05π/amomentum range centred on the SDW gap for each temperature) as inFig. 2cfrom aboveTS/TSDWto belowTC. Each EDC is fitted with two Lorentzians and a linear background, with the fit shown by the black curve. Diamonds indicate the peak positions above and below the SDW gap, where the error bars indicate the standard deviations from the fits. Shaded region indicates the effective SDW gap as a function of temperature. (b) Symmetrized EDCs at thekFpoint of the band crossing as inFig. 2c, for temperatures acrossTC. Diamonds indicate lower branch of the SDW gap, circles indicate superconducting peaks. Black lines are symmetrized fits to the symmetrized EDCs with the Norman model34for the SC gap, a Lorentzian for the SDW peak, and a second order polynomial for the background. (c) The extracted effective SDW gap size for the undoped (black) and UD compound (red), along with the extracted SC gap size for the UD compound (blue), as a function of temperature. The error bars are from the properly combined s.d. of the fitted positions of the two peaks in each EDC marking the upper and lower edges of the SDW gaps. Figure 4: Temperature dependence of the SDW and SC gaps. ( a ) EDCs divided by Fermi–Dirac function convolved with a Gaussian representing instrumental resolution taken across the SDW gap (integrated EDCs within a Δ k x =0.05π /a momentum range centred on the SDW gap for each temperature) as in Fig. 2c from above T S / T SDW to below T C . Each EDC is fitted with two Lorentzians and a linear background, with the fit shown by the black curve. Diamonds indicate the peak positions above and below the SDW gap, where the error bars indicate the standard deviations from the fits. Shaded region indicates the effective SDW gap as a function of temperature. ( b ) Symmetrized EDCs at the k F point of the band crossing as in Fig. 2c , for temperatures across T C . Diamonds indicate lower branch of the SDW gap, circles indicate superconducting peaks. Black lines are symmetrized fits to the symmetrized EDCs with the Norman model [34] for the SC gap, a Lorentzian for the SDW peak, and a second order polynomial for the background. ( c ) The extracted effective SDW gap size for the undoped (black) and UD compound (red), along with the extracted SC gap size for the UD compound (blue), as a function of temperature. The error bars are from the properly combined s.d. of the fitted positions of the two peaks in each EDC marking the upper and lower edges of the SDW gaps. Full size image The coexistence of magnetism and SC holds a special fascination in the field of HTSC as magnetism is generally believed to be detrimental to SC [29] , [30] . Extensive efforts have been made to understand whether this coexistence in the pnictides is indeed microscopic as it would have strong implications on the mechanism of SC in these compounds. In particular, theoretical work has shown that a conventional s ++ pairing symmetry state cannot coexist with the SDW order, whereas such coexistence is possible for an unconventional s ± pairing symmetry [31] . Using a simple simulation of the APRES spectra, we show that our observation of the reduced SDW gap and its shift towards E F as well as the observation of a well-defined superconducting gap below T C on the same spectrum cannot be explained by a phase-separated coexistence of these orders but more consistent with a microscopic coexistence scenario ( Supplementary Note 5 ), in agreement with NMR measurements [32] , pointing to s ± pairing symmetry for this part of the phase diagram. Furthermore, it is clear from our results that the SDW and nematic orders are not mere spectators to the presence of SC. The SDW gap—a representation of the strength of the coherent electronic excitations of the SDW order—is suppressed with the onset of SC, indicating that the SDW order competes with SC for the same electrons. The fact that a reduction in both Δ SDW and Δ S is required to fully account for the experimental observations also demonstrates that the SDW order and the electronic nematicity are intimately connected and both are likely in competition with SC in the coexistence region. Lastly, it is interesting to point out the connection to the cuprates. Traditionally, there have been two main interpretations of the PG phase: (i) a precursor state of SC, (ii) a competing phase to SC. While several recent reports favour the scenario of competition [1] , [2] , [3] , [4] , the elusive nature of the PG complicates the interpretations. Here, we demonstrate clearly with spectroscopic evidence the competition between SC and a well-characterized long-range density wave, which is intriguingly similar to a recent study in cuprates showing a similar suppression of the PG spectral features associated with the onset of SC (M. Hashimoto et al. submitted). While the competition in iron pnictides may be simpler than that in the cuprates, the comparison of the two families may provide helpful insights on the mysterious PG phase in the cuprates, and help link the two families for an eventual understanding of the mechanism of unconventional SC. Experimental conditions High-quality single crystals of Ba 1− x K x Fe 2 As 2 were grown using the self-flux method [18] . Mechanical detwinning of the crystals was performed using a previously reported method [9] . ARPES measurements were carried out at both beamline 5-4 of the Stanford Synchrotron Radiation Lightsource and beamline 10.0.1 of the Advanced Light Source using SCIENTA R4000 electron analysers. The total energy resolution was set to 5 meV and the angular resolution was 0.3°. Single crystals were cleaved in situ below 10 K for each measurement. All measurements were done in ultra high vacuum with a base pressure lower than 4 × 10 −11 torr. Tight-binding model simulations The simulations used in Fig. 3 were produced based on a five-orbital tight-binding model of BaFe 2 As 2 from DFT band structure [24] . The E F was first shifted down by 0.15 eV to account for the hole doping. The bands were then renormalized by a factor of 3 to match the observed band structure for the UD compound. The cut of the calculations shown in Fig. 3 was along k y =0.07π/ a , to match the experimental cut shown in Fig. 2 . The parameters used in Fig. 3 were implemented as described in the following. The orbital anisotropy, Δ S , is an onsite energy splitting between d xz and d yz that is momentum dependent ( Δ S ( k )=α·sin 2 ((| k x |+| k y |)/2), which is zero at Γ and maximum at X / Y along the high-symmetry directions, and also periodic in k , see Supplementary Note 1 ), where α{d xz , d yz }={−20 meV, 40 meV}. The SDW order parameter, Δ SDW , is diagonal in the orbital basis, with Δ SDW {d xz , d yz , d x 2− y 2 , d xy , d 3 z 2−r2 }=30 meV*{0.25, 1, 0.25, 0.5, 0.25}. The ratios between the different orbitals are consistent with the results of self-consistent calculations for the SDW order in the orbital basis, in which d yz bands tend to open the largest SDW gap [33] . The superconducting order parameter, Δ SC , is taken to be isotropic and 5 meV. How to cite this article: Yi, M. et al. Dynamic competition between spin-density wave order and superconductivity in underdoped Ba 1− x K x Fe 2 As 2 . Nat. Commun. 5:3711 doi: 10.1038/ncomms4711 (2014).